Spectral non-uniform temperature and non-local heat transfer in the spin Seebeck effect Recently discovered spin-dependent thermoelectric effects have merged spin, charge, and thermal physics, known as spin caloritronics, of which the spin Seebeck effect is its most puzzling. Here we present a theory of this effect driven by subthermal non-local phonon heat transfer and spectral non-uniform temperature. The theory explains its non-local behaviour from the fact that phonons that store the energy (thermal) and the phonons that transfer it (subthermal) are located in different parts of the spectrum and have different kinetics. This gives rise to a spectral phonon distribution that deviates from local equilibrium along the substrate and is sensitive to boundary conditions. The theory also predicts a non-magnon origin of the effect in ferromagnetic metals in agreement with observations in recent experiments. Equilibration of the heat flow from the substrate to the Pt probe and backwards leads to a vertical spin current produced by the spin-polarized electrons dragged by the thermal phonons. The key and most intriguing effect in spin caloritronics [1] , [2] , [3] , [4] , [5] , [6] , [7] , [8] , [9] is the transverse spin Seebeck effect (SSE) in which a thermal gradient in a ferromagnet/substrate structure gives rise to spin currents that vary along the length of the sample and are detected via the inverse spin-Hall voltage [10] . This effect has been experimentally observed using different ferromagnetic materials: metals [1] , semiconductors [2] , [3] and insulators [4] . The magnitude of the SSE is quantified by the transport coefficient , where V y is the measured ISHE voltage, w is the width of Pt probe, and x T =( T 2 − T 1 )/ L , where L is the length of the sample, see Fig. 1a . The ISHE voltage is given by , where j s is the spin current, s is its polarization, θ H is the spin-Hall angle of the probe (in Pt, θ H is of the order of one per cent) and ρ is its electric resistivity. The effect is non-local, that is, it depends on the position along the sample rather than the local temperature gradient. In addition, the size of the sample is usually about 1 cm and such a long-range information about position can be transferred only by phonons, propagating along the insulating substrate [2] . The key role of phonons for the transversal SSE effect was discussed in Adachi et al. 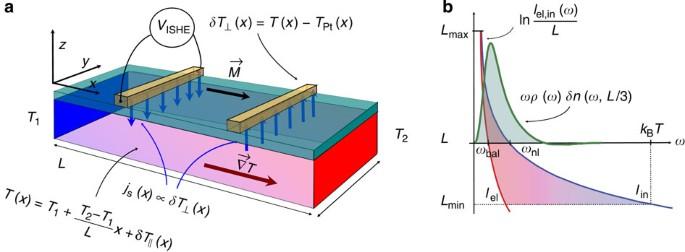Figure 1: Scheme of the SSE experiment. (a) The effect incorporates three key physical mechanisms: (i) subthermal phonons whose inelastic length,lin, is of the order of the sample size,L, and whose elastic length,lel, is smaller thanL, drive the non-local heat propagation along the substrate, which gives rise to a steady-state distribution function that deviates from local equilibrium; (ii) equilibration of heat flows out of the substrate into the Pt probe and backwards establishes the temperature in the probeTPt≠T(x); (iii) the different phonon distribution functions in the probe and the substrate yield a spin-phonon-drag current,. (b) Spectral phase diagram of phonons as a function of sample length. The deviation from local thermal equilibrium, δn(ω,x)=n(ω,x)−nT(x)(ω), is illustrated (green curve) forx=L/3; hereρph(ω)ω2is the phonon density of states. [5] Figure 1: Scheme of the SSE experiment. ( a ) The effect incorporates three key physical mechanisms: (i) subthermal phonons whose inelastic length, l in , is of the order of the sample size, L , and whose elastic length, l el , is smaller than L , drive the non-local heat propagation along the substrate, which gives rise to a steady-state distribution function that deviates from local equilibrium; (ii) equilibration of heat flows out of the substrate into the Pt probe and backwards establishes the temperature in the probe T Pt ≠ T ( x ); (iii) the different phonon distribution functions in the probe and the substrate yield a spin-phonon-drag current, . ( b ) Spectral phase diagram of phonons as a function of sample length. The deviation from local thermal equilibrium, δ n ( ω , x )= n ( ω , x )− n T ( x ) ( ω ), is illustrated (green curve) for x = L /3; here ρ ph ( ω ) ω 2 is the phonon density of states. Full size image Here we show that the non-locality of the SSE is a consequence of the non-local energy transfer due to subthermal diffusive phonons that are sensitive to the boundary conditions and give rise to a spectral non-uniform temperature along the sample [11] , [12] . In fact, in recent measurements in bilayer F–Pt wire devices, the specific geometry excludes long-ranged propagation of magnons and leaves only phonons as a source of non-locality [6] . In addition, we demonstrate that while in the insulator the SSE is likely determined by the phonon–magnon mechanism, in the conducting ferromagnet (for example, Ni 81 Fe 19 (ref. 1 ) and GaMnAs [3] ), the magnon mechanism is not the only one available. The experiments by Jaworski et al. [3] were performed on a material with Curie temperature T C =130 K, considerably lower than the Debye temperature θ D =350 K, and showed that V ISHE M at the vicinity of the Curie point; that is, the SSE signal vanishes with the magnetization M with the same critical behaviour. This latter fact excludes the magnon mechanism for this case: as we have checked, starting from equation 12 of Adachi et al. [13] , the magnon pumping yields the contribution to the SSE signal, which vanishes as M 3/2 (see Supplementary Note 1 for details). Physical mechanisms of the phonon–electron SSE The theory of this phonon–electron SSE, which does not involve magnons, has three key physical mechanisms. The first (i) involves the non-local nature of the signal driven by subthermal phonons, which is also relevant for the magnon-phonon mechanism not considered here. In recent measurements of the SSE in insulators [14] , the temperature difference between thermal magnons and phonons assumed in the current theory [13] , [15] has not been observed, suggesting the necessity of the concept of spectrally non-uniform temperature. This concept originates from the fact that in most dielectrics, and also some semiconductors, the energy transfer is highly non-local [11] , [12] because of the strong dependence of the diffusion coefficient of phonons on frequency: D ( ω ) ω −4 , if the dominant scatterers are point-like [16] . In the diffusive regime of the experiments the energy relaxation length is given by where the energy relaxation rate is While the thermal phonons, ħ ω ~ k B T , are equilibrated, the subthermal low-frequency phonons can deviate from the local equilibrium due to the rapid low-frequency growth of inelastic length l in ( ω )= l in ( T )( T / ω ) 5/2 , which leads to non-local kinetics. Even the concept of temperature itself is well defined only for phonons of high-enough frequency. For the ‘thermal’ part of the spectrum ħ ω ≥ k B T , the distribution function has a Planckian form n T ( ω )=( e ℏ ω / k B T − 1 ) −1 with a local temperature T = T ( x ). As a result, the phonons that store the energy and phonons that transfer it are located in different parts of the spectrum. As illustrated in Fig. 1b , this spectral separation occurs when l el ( T )<< l in ( T )<< L , where l el ( T )≡ l el (ħ ω = k B T ) D (ħ ω = k B T ) T −4 , and l in ( T )≡ l in (ħ ω = k B T ) T −4.5 . Then the subthermal phonons whose inelastic length is of the order of (but whose elastic length is much shorter) than L drive the non-local heat propagation along the substrate, giving rise to a steady-state phonon distribution function that deviates from local equilibrium for ħ ω << k B T and depends on the position along the substrate. This deviation from local thermal equilibrium in the low frequencies manifest in a T ( x ) profile that deviates from a linear dependence. To describe this non-local effect, it is essential to formulate the boundary conditions for the equations describing the propagation of the diffusive phonons. (Previously [15] , the sensitivity to the boundaries entered the theory as a result of the different boundary conditions imposed on phonons and magnons [17] . This model, however, cannot explain the position dependence of the SSE signal, measured on the sample with a scratched magnet [2] or on the bilayer wire device [6] . Here, instead, we demonstrate that phonons in different parts of the energy spectrum act as the ‘subsystems’ of different sensitivity to the boundaries). The second (ii) mechanism involves the electron–phonon drag. As the probe is a ‘dead end’, there is a full balance between incoming and outgoing heat fluxes such that net heat flux is zero. However, the incoming and outgoing fluxes have different spectral distributions, because of the inelastic processes in Pt, which average out the spectrum of the incoming flux, and establish a local temperature T Pt ( x ) different from T ( x ). The spin drag, induced by the phonon flux, is sensitive to the spectral content of the phonon distribution function. Hence, despite zero net heat flux, the spin injection is not zero. In the stationary situation, the drag voltage induced by the phonons is compensated by redistribution of the electron density, so that the total electric current is zero (as well as electrochemical potential gradient). However, in the presence of a spin polarization, there will be a net spin current j s = j ↑ − j ↓ polarized along magnetization M : unlike its charge counterpart, spin drag is not blocked by accumulation of the spin density, which is eliminated by the SO interaction in Pt. The magnitude of j s depends on the ratio of the thickness of the ferromagnet, d F , and the phonon inelastic scattering length there, . The optimal value of d F for observing the phonon drag SSE is of the order of . For too thin ferromagnet, , the phonons cannot effectively transfer their momentum to electrons to drag them towards the probe. In the opposite limit, , the phonons equilibrate before they reach the region near the probe. An alternative mechanism not considered here is the quantum acoustoelectric pumping [18] due to the spectrally non-uniform flux of phonons (O. Tretiakov, K.S.T., J.S., A.M.F., manuscript in preparation). The final (iii) mechanism involves the conversion of the spin current to an electric signal via the ISHE. This conversion is most optimal if the thickness of the Pt layer is of the same order of magnitude as the spin relaxation length in Pt, which is the case in the discussed experiments [19] . As shown in detail in the following sections, the resulting theory gives the correct magnitude of the signal, predicts a dependence on magnetization S SSE M , and gives specific temperature and size dependencies that can be tested experimentally. Subthermal phonon kinetics On Fig. 1b , we show the spectral phase diagram of frequency regions contributing differently to the kinetics of phonons. There are two characteristic frequencies, ω nl and ω bal , determining the propagation of phonons: For non-local transport, we require ħ ω nl = k B T ( L / l in ( T )) −2/5 << k B T . In addition, we will not be interested in phonons in the ballistic part of the spectrum, ω < ω bal . This is legitimate as long as ω bal << ω nl , and determines a maximum length of the sample, L max , given by the point of intersection of the curves l in ( ω ) and l el ( ω ), as shown in Fig. 1b . This gives a temperature dependence L max T − 16/3 . For lengths larger than L max , the non-local effect is due to the fraction of phonons propagating ballistically and requires a different formalism, which we will not discuss here. The other condition that allows to separate thermal phonons from those which produce non-local effects is l in ( T )<< L . This gives a minimum length of the sample L min T − 9/2 . For length smaller than L min even thermal phonons are out of equilibrium and spectral separation does not hold. The large ratio of l in ( T )/ l el ( T ) opens the window which we are interested in. Hence, the sample size should be in the range indicated on Fig. 1b . Estimation at T =10 K (when typical phonon energy is 28 K), gives L max about few centimetres and L min on the scale of milimetres. Recall that the typical size of the sample used for the SSE experiments is 1 cm. With temperature, the width of the region of applicability of the theory behaves as L max / L min T −5/6 and we expect it to be relevant up to 50 K. In addition, the temperature is assumed to be much smaller than the Debye temperature, T << θ D , which allows us to ignore Umklapp processes. With these specific length restrictions, we consider next the theory of propagation of diffusive phonons along the substrate. Owing to the fact that the low-frequency phonons do not primarily interact with themselves but with equilibrated high-frequency phonons, one may use the following kinetic equation that describes propagation of phonons in the insulating substrate, valid for ħ ω ≲ k B T : where δ n is the deviation from the local equilibrium The solution to this second-order differential equation requires two sets of effective boundary condition equations. The first, which establishes T ( x ) from a given δ n ( x , ω ), is obtained from continuity of the energy density in the system, which in stationary situations reads as . Because of the divergence of D ( ω ) at small ω , the heat flux is transported by the low-energy part of the spectrum [20] , [21] , [22] . The heat current density is given by: where ρ ph ( ω ) ω 2 is the phonon density of states (summed over all branches). The integral for diverges and has to be cutoff at small frequency (the exact value of the cutoff does not enter our results, as the integral for converges). Using equation (2), the energy density continuity equation takes the following form: This equation should hold for all x . Thus, one has to solve a system of integro-differential equations. For the case of a pulse propagation in an infinite media, the non-local phonon transport has been studied in Levinson [11] , [12] and Wilson and Schaich [23] . However, we are interested in a stationary solution in the presence of the boundaries which yield the second equation that fully establishes n ( ω,x ) and T ( x ). On the boundary between the substrate and the heater, there is a jump in the phonon distribution function because of the abrupt change in the properties of materials. This leads to a finite thermal boundary resistance (Kapitza resistance), which manifests itself through the jump Δ T K at the contact [24] . If the scattering in the vicinity of the boundary is mostly elastic, the boundary condition consists of conservation of spectral heat current density across the boundary. It relates the heat flux through the boundary to the jump of the phonon distribution function across it. At the left end of the sample (which is at heat contact with a reservoir at temperature T 1 ) it takes the following form: The boundary resistance R Bd is assumed to be frequency independent. If the heat contacts are in thermal equilibrium, R Bd can be related to the thermal boundary conductivity where v s is the averaged sound velocity. Note, that in the absence of the boundary resistance ( R Bd =0), the locally equilibrated distribution function n ( ω , x )= n T 0 ( x ) ( ω ) with T 0 ( x )= T 1 +( T 2 − T 1 ) x / L satisfies the kinetic equation, so that δ n =0 and the non-local effect vanishes, as the boundaries are effectively at infinity. One may easily see that δ n R Bd at not too large values of R Bd . With this it is then possible to write down a closed equation for T ( x ). If the phonon temperature as a function of position x is known, the distribution function can be obtained from equation (2) and reads: where x < =min ( x , x ′), x > =max ( x , x ′). The ‘source’ term n S ( ω , x ) comes from the boundary condition (equation (6)) and is equal to where and Above we have introduced the effective boundary thermal conductance . The second term in equation (7) describes the process of redistribution of phonons along the sample due to diffusion and inelastic scattering. Substituting equation (7) into equation (5), one gets an integral equation for T ( x ), which can be solved numerically. This procedure is self-consistent: after finding T ( x ), the distribution function is easily calculated from equation (7). To illustrate the result, we assume the following ratios of characteristic lengths of a thermal phonon and calculate the correction to the linear temperature behaviour which is shown on Fig. 2 , where we have assumed that R Bd =0.1 and T 1 < T 2 . Although the deviation from the linear behaviour is small, it ensures the conservation of the energy density of the phonons propagating along the substrate. Ultimately, the non-equilibrium correction δ n ( ω , x ) is responsible for the SSE effect. In Fig. 1b , the frequency dependence of ħ ωρ ph ( ω )δ n ( ω , x ) is plotted close to the colder end (for x =0.3 L ). On the hotter end, δ n has the opposite sign. 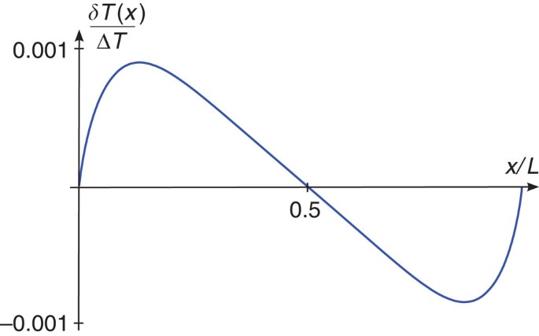Figure 2: Correction to temperature behaviour. Correction to the linear temperature dependence as a function of position, equation (12). Figure 2: Correction to temperature behaviour. Correction to the linear temperature dependence as a function of position, equation (12). Full size image Out-of-plane spin transport After finding the non-equilibrium distribution function of phonons δ n ( ω , x ), we next concentrate on the heat and spin transport in the vertical direction from the substrate to the probe across the magnet. The temperature of phonons in the Pt probe, T Pt ( x ), is different from the T ( x ). It is determined by the requirement that the heat flux created by non-equilibrium non-local phonons from the substrate to Pt is compensated by backflow flux of thermal phonons from Pt to the substrate. The resulting temperature difference, δ T ┴ ( x )= T ( x )− T Pt ( x ), can be found from the heat balance equation: where δ N ( ω , x )= n sub − n Pt is the difference of the distribution function of phonons entering and leaving the Pt probe, located at x . Here we neglect inelastic scattering of phonons while they pass through the ferromagnetic layer ( ), and have assumed the sound velocities to be of similar order in the Pt and the substrate. We also assume, that the probe is small enough a << l el ( T ), so that the influence of the counterflow on the phonon distribution function in the substrate can be ignored. It is useful to present δ N ( ω , x ) in the following form: Then, the temperature difference δ T ┴ ( x ) can be calculated from the equation: where h ( x ) is the dimensionless heat flux supplied to the probe by the non-equilibrium phonons. The function h ( x ) can be written in a form of where H ( x ) is a slow function of temperature and boundary resistance R Bd . Here ω bal encodes information about scattering of phonons on the disorder and the length of the sample. Function H ( x ) is plotted on Fig. 3 for the same sample parameters as before. 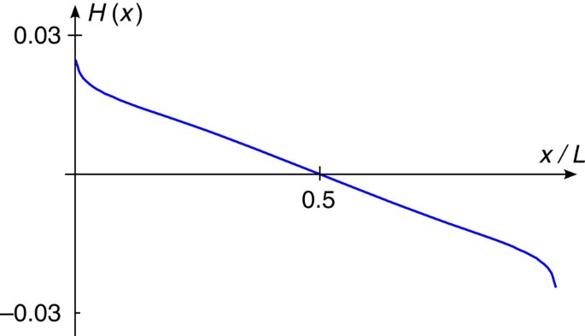Figure 3: The function of temperature and boundary conditionsH(x). The functionH(x)δT┴(x) determining the magnitude and spatial profile of the SSE signalSxygiven in equation (20). Figure 3: The function of temperature and boundary conditions H ( x ). The function H ( x ) δ T ┴ ( x ) determining the magnitude and spatial profile of the SSE signal S xy given in equation (20). Full size image With this we can finally estimate the scale of the SSE due to conducting electrons, dragged by out-of-equilibrium phonons, in more detail. The guiding idea about the scale of the effect follows from the derivation of the well-known Gurevich formula [25] , [26] , [27] for the phonon drag. This formula gives for thermoelectric coefficient η =− j / T the following expression: , which is valid when q T l >>1 (here q T = k B T /ħ v s is the wavevector of a thermal phonon). For the dirty case q T l <<1, the particle current density dragged to the probe is given by Sergeev and Mitin [28] : We write τ ei , l ei for electron-impurity scattering time and length in the ferromagnet. The role of electron-impurity scattering in equation (16) is twofold. It enhances electron–phonon interaction by slowing the motion of electrons (making it diffusive). This is taken into account by the form of W ( x ). On the other hand, it diminishes the drag effect due to the loss of electron momentum by impurity scattering. The details of the function W ( x ) depend on the character of the scattering of phonons on defects. We assume that phonons scatter on impurities vibrating with the lattice [29] and W ( x )= W vb ( x ). For temperatures k B T <<ħ v s / l ei , we may use the asymptotic behaviour W vb ( x <<1)≈ x . Recalling that the charge current will be compensated by an unpolarized backflow charge current from the Pt probe, the total spin current is given by the polarized current dragged by the phonons into the Pt probe. Finally, we rewrite the expression for the spin-phonon-drag current injected into the Pt probe as where A el ( T )=( k B T / ε F ) ( k F l ei ) 2 is a dimensionless constant, determined by electrons, is the level of spin polarization and the dragging factor is As the spectral densities of the energy and the charge currents are proportional to different powers of the phonon frequency, the electronic drag due to phonons is possible even when the net energy flow is zero. The contribution to J in equation (18) arising due to the temperature difference δ T ┴ ( x ) between the substrate and the Pt probe (first term in equation (14)) is dominant. In other words, while the non-locality of the effect along the sample is carried by the low-frequency phonons, the dragging force generating the spin current is produced by the thermal phonons. As a result of this intricate joint effort by the phonons in different parts of the spectrum, one gets (restoring units): Finally, for the magnitude of the SSE, , and recalling that δ T ↑ ( x ) − Th ( x ), we obtain: where is a material-dependent constant. The factor 2.8 takes into consideration that the energy of thermal phonon is 2.8 k B T . Assuming that in Pt, ρ =0.9 μΩ· m and , we obtain . Function H ( x ) is positive at the cold end, meaning the dragging force pushes electrons towards the magnet there, according to equation (19). Note that although the electron–phonon drag is proportional to a high power of temperature, see equation (17), the final result for the SSE coefficient is only weakly temperature dependent, S xy T . It comes out as a result of the strong dispersion of the phonon-scattering time in the substrate. Although function H ( x ) in equation (20) is also temperature dependent, this dependence comes only from the non-locality of the phonon collision integral in energy, and is relatively weak. Another important property of this function is that its spatial profile varies with temperature rather slowly. This is because the phonons which contribute mostly to the non-local effect have inelastic scattering length of the order of the sample size. Varying the temperature mainly results in the shift of the relevant phonon energy ω nl , so that the corresponding length scale l in ( ω nl ) remains the same. These observations stress the importance of the strong dispersion of the phonon scattering. Taking θ H =0.08, ε F / k B =10 3 K, θ D =350 K, k F l ei =10 and the ratio of characteristic lengths as in equation (11), we find the magnitude of the effect at 10 K to be S ~20 μV K −1 × X M . In this work, we have discussed the main ingredients of the phonon dynamics in the substrate that allows to understand the spatial profile of the SSE signal. As we have shown, to explain the non-local effect, i.e., its dependence on the position of the probe along the substrate, one must consider the spectral non-uniformity of the phonon distribution function, which can be interpreted as spectrally non-uniform temperature. A key aspect of the non-locality is the explicit introduction of the boundaries into the equations describing the propagation of diffusing phonons. In addition, we have presented a scheme of the non-magnon mechanism in the case when the ferromagnetic element of the device is conducting and obtain the correct magnitude of the effect. (The recent observation [30] of the magnetic proximity effect in FM/Pt contact suggests the possibility of another channel to contribute to the SSE voltage: anomalous Nernst effect. However, it is less universal than the electron–phonon drag and in any case must rely on the mechanism, which we propose for generation of the non-local signal: subthermal phonons with energy-dispersive diffusion, which is quite universal.) Furthermore, the spatial profile of the SSE signal, presented in Fig. 3 , is very similar to the one shown as a ‘universal’ profile on the figure 2f of Jaworski et al. [2] Although the phonon kinetics at temperatures comparable with θ D is strongly modified by Umklapp processes, the measured proportionality between the SSE signal and the magnitude of the magnetization in Jaworski et al. [3] clearly indicates that near T C ≈130 K, the effect is still dominated by the flux of the spin-polarized electrons, instead of the magnon-mediated spin torque. We believe that the difference between the data presented in figures 2 and 3 of Jaworski et al. [3] — in particular, the difference in the behaviour near the T C ,—supports this picture. Two different samples demonstrate drastically different temperature behaviour. The sample that is thicker and grown on a substrate of a better quality has larger peak value of both S xy and thermopower α xx and also much faster decay of S xy at approaching T C . The stronger thermopower observed in the thicker sample demonstrates that in this sample, phonons lose momentum mainly in collisions with electrons, while in the thinner sample, their scattering on the defects is more efficient. However, due to strong sensitivity of the phonon distribution function at the F–Pt boundary to the ratio , in the thicker sample, the SSE decays with temperature much faster than in the thinner one. As we have already discussed, at large , the phonons equilibrate before they reach the probe. Indeed, in the thicker sample (more than three times thicker than the thinner one), the effect was not even resolved near the Curie temperature within the accuracy of the measurement. This suggests the need to study the dependence of the SSE signal on the thickness of the magnetic sample in otherwise identical conditions, that is, keeping the properties of the insulating substrate and semiconductor/substrate boundary the same. How to cite this article: Tikhonov, K. S. et al. Spectral non-uniform temperature and non-local heat transfer in the spin Seebeck effect. Nat. Commun . 4:1945 doi: 10.1038/ncomms2945 (2013).